The FAM3 superfamily member ILEI ameliorates Alzheimer’s disease-like pathology by destabilizing the penultimate amyloid-β precursor Accumulation of amyloid-β peptide (Aβ) in the brain underlies the pathogenesis of Alzheimer’s disease (AD). Aβ is produced by β- and γ-secretase-mediated sequential proteolysis of amyloid-β precursor protein (APP). Here we identify a secretory protein named interleukin-like epithelial-mesenchymal transition inducer (ILEI, also known as FAM3 superfamily member C) as a negative regulator of Aβ production. ILEI destabilizes the β-secretase-cleaved APP carboxy-terminal fragment, the penultimate precursor of Aβ, by binding to the γ-secretase complex and interfering with its chaperone properties. Notch signalling and γ-secretase activity are not affected by ILEI. We also show neuronal expression of ILEI and its induction by transforming growth factor-β signalling. The level of secreted ILEI is markedly decreased in the brains of AD patients. Transgenic (Tg) overexpression of ILEI significantly reduces the brain Aβ burden and ameliorates the memory deficit in AD model mice. ILEI may be a plausible target for the development of disease-modifying therapies. The amyloid-β peptide (Aβ) is produced in neurons by two-step proteolytic processing of the amyloid-β precursor protein (APP) [1] . Ectodomain shedding by β-secretase, which is known as β-site APP-cleaving enzyme 1 (BACE1), yields the membrane-spanning carboxy-terminal fragment (CTF)-β. The aspartyl protease γ-secretase complex, which primarily comprises presenilin, nicastrin (NCT), anterior pharynx defective-1 (APH-1) and presenilin enhancer-2 (PEN-2), sequentially catalyses intramembrane proteolysis of APP-CTFβ, resulting in secretion of Aβ and liberation of the APP intracellular domain [1] . Each proteolysed derivative exhibits distinct physiological activities [2] , and genetic ablation of APP in mice causes neurological deficits such as impairment of spatial learning and reduction in brain weight, which can be completely rescued by expression of the secreted ectodomain [3] . Ablation of the γ-secretase complex by genetic deletion of any of the core components causes early developmental defects that resemble a Notch phenotype, which is expected because γ-secretase is involved in transmembrane signal transduction by cleaving various membrane-spanning substrates, including Notch receptors [1] . A persistent imbalance between production and clearance of Aβ results in gradual accumulation of soluble and aggregated Aβ in the extracellular space of the brain parenchyma, which underlies the development of Alzheimer’s disease (AD). Genetic mutations in APP, presenilin-1 (PS1) and presenilin-2 (PS2) modify Aβ biosynthesis and cause an autosomal dominant form of AD [4] . In contrast, alteration in Aβ metabolism in the common sporadic form of AD has not been fully clarified. However, an increase in the amount and activity of BACE1 and/or a decline in protein degradation capacity have been proposed as the primary events in the pathogenesis of sporadic AD [5] , [6] , [7] , [8] . In addition to Aβ, accumulation of APP-CTFs, which are sometimes associated with sporadic AD, may cause neurodegeneration by inducing abnormal membrane currents, decreased numbers of dendritic spines, neuronal cell death and inflammatory reactions [9] , [10] . Reduction in brain Aβ is the pivotal goal of disease-modifying therapy for AD. Although γ-secretase is a major target for therapeutic intervention, non-selective inhibition of its activity causes serious adverse effects due to blockade of Notch signalling and accumulation of neurotoxic APP-CTFs [1] , [11] , [12] , [13] . To avoid these adverse effects, finding novel approaches to negatively modulate Aβ generation is imperative. Several endogenous proteins interact with the γ-secretase complex and influence the efficacy of γ-secretase cleavage in distinct ways, including alteration of specific activities, substrate selectivity and assembly or subcellular localization of γ-secretase complexes [14] , [15] , [16] , [17] . In this study, we searched for additional proteins that affect Aβ generation by interacting with the γ-secretase complex. To date, multiple γ-secretase-modulating proteins have been identified by purification of intact γ-secretase complexes via affinity-mediated isolation of the major catalytic component, PS1 (refs 18 , 19 ), which is also involved in cellular Ca homeostasis, apoptosis and protein trafficking by binding additional or alternative partners [14] . In contrast, PEN-2 is exclusively involved in formation of the γ-secretase complex, as the cellular accumulation of PEN-2 is entirely dependent on the expression of the other core components. In addition, PEN-2 is the last component to be incorporated into the γ-secretase complex, and activated complexes exclusively contain PEN-2. Here, using PEN-2 affinity-mediated isolation of the γ-secretase complex, we identify a unique secretory protein that reduces cellular Aβ generation without inhibiting γ-secretase activity or Notch cleavage. ILEI is a γ-secretase complex-binding protein We employed tandem affinity-tag purification (TAP) [20] to isolate the γ-secretase complex using PEN-2 as the bait, combined with stable silencing of endogenous PEN-2 expression. The abundance and stoichiometry of γ-secretase components are tightly regulated. Although exogenous PEN-2 can be incorporated into the γ-secretase complex by replacing endogenous PEN-2, high PEN-2 overexpression is required for sufficient replacement. To circumvent this problem, we first prepared PEN-2-knockdown HEK293 cell lines in which small interference RNA (siRNA) for PEN-2 was stably expressed. We chose a PEN-2-knockdown cell line that exhibited the lowest levels of PEN-2 expression and Aβ secretion. We then transfected this cell line with siRNA-resistant PEN-2 (srPEN-2) fused with a TAP tag (TAP-srPEN-2) and selected a cell line, referred to as HEK-TAP-PEN-2, which stably expressed TAP-srPEN-2 at a level equivalent to that of endogenous PEN-2. We confirmed that TAP-srPEN-2 was incorporated into the active γ-secretase complex and restored Aβ secretion ( Supplementary Fig. 1 ). The activity and composition of γ-secretase complexes are sensitive to several detergents but are only slightly affected by 1% 3-[(3-cholamidopropyl)dimethylammonio]-2-hydroxy-1-propanesulfonic acid (CHAPSO) [21] . We prepared CHAPSO lysates of HEK-TAP-PEN-2 cells and performed sequential isolation of TAP-srPEN-2-associated complexes. To distinguish non-specific binding proteins from proteins of interest, we used TAP-tag-transfected PEN-2-knockdown HEK293 (HEK-TAP-empty) cells as a control. Complexes isolated in two independent trials exhibited a similar pattern of banding on SYPRO- and silver-stained SDS–polyacrylamide gel electrophoresis (SDS–PAGE) gels ( Fig. 1a ). Proteins in each excised gel piece were digested with trypsin and subjected to liquid chromatography-tandem mass spectrometric analysis followed by a search of the Mascot database. Hits included the four core components and some known binding proteins of the γ-secretase complex. One of the identified peptides matched residues 164–179 of a 27-kDa protein referred to as interleukin-like epithelial-mesenchymal transition inducer (ILEI) or family with sequence similarity 3, member C (FAM3C) (NCBI Protein Database accession code NP_055703). 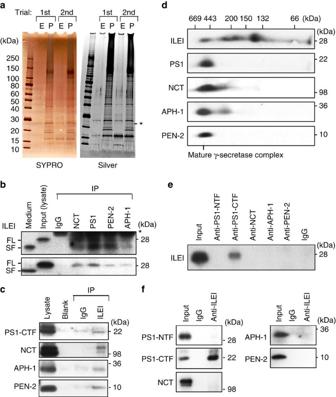Figure 1: ILEI is associated with mature γ-secretase complexes. (a) SYPRO- and silver-stained SDS–PAGE gels of TAP-tagged PEN-2-associated proteins isolated from lysates of HEK-TAP-PEN-2 (P) and HEK-TAP-empty (E) cells. ILEI was identified in the band indicated by the star. (b) Co-immunoprecipitation of endogenous ILEI and γ-secretase components. Native HEK293 cell lysates were immunoprecipitated with normal IgG or an antibody against NCT, PS1, PEN-2 or APH-1. The blot was probed with anti-ILEI antibody (upper panel). As the FL ILEI bands were close to the IgG light-chain bands, nanocapsules incorporating IgG Fc-binding Z domains were used instead of the secondary antibody for detection (lower panel). The star indicates the IgG band. FL, full-length; SF, secreted form. (c) Reverse co-immunoprecipitation. HEK293 cell lysates were precipitated using normal rabbit IgG (IP-IgG) or anti-ILEI antibody (IP-ILEI). The blots were probed using the indicated antibodies. (d) Two-dimensional Blue Native (BN)/SDS–PAGE analysis of ILEI and γ-secretase components. The membrane fraction of native HEK293 cells was subjected to two-dimensional BN/SDS–PAGE before immunoblotting. (e) Chemical crosslinking of ILEI with γ-secretase components. HEK293 cells were crosslinkedin situwith dithiobis succinimidyl propionate. The 1% Nonidet P-40-solubilized cell lysate was subjected to immunoprecipitation. A blot of the immunoprecipitates with antibodies against the indicated proteins or normal IgG was probed with anti-ILEI antibody. (f) The crosslinked cell lysates were immunoprecipitated using normal IgG or anti-ILEI antibody. The blots were probed using the indicated antibodies. Figure 1: ILEI is associated with mature γ-secretase complexes. ( a ) SYPRO- and silver-stained SDS–PAGE gels of TAP-tagged PEN-2-associated proteins isolated from lysates of HEK-TAP-PEN-2 (P) and HEK-TAP-empty (E) cells. ILEI was identified in the band indicated by the star. ( b ) Co-immunoprecipitation of endogenous ILEI and γ-secretase components. Native HEK293 cell lysates were immunoprecipitated with normal IgG or an antibody against NCT, PS1, PEN-2 or APH-1. The blot was probed with anti-ILEI antibody (upper panel). As the FL ILEI bands were close to the IgG light-chain bands, nanocapsules incorporating IgG Fc-binding Z domains were used instead of the secondary antibody for detection (lower panel). The star indicates the IgG band. FL, full-length; SF, secreted form. ( c ) Reverse co-immunoprecipitation. HEK293 cell lysates were precipitated using normal rabbit IgG (IP-IgG) or anti-ILEI antibody (IP-ILEI). The blots were probed using the indicated antibodies. ( d ) Two-dimensional Blue Native (BN)/SDS–PAGE analysis of ILEI and γ-secretase components. The membrane fraction of native HEK293 cells was subjected to two-dimensional BN/SDS–PAGE before immunoblotting. ( e ) Chemical crosslinking of ILEI with γ-secretase components. HEK293 cells were crosslinked in situ with dithiobis succinimidyl propionate. The 1% Nonidet P-40-solubilized cell lysate was subjected to immunoprecipitation. A blot of the immunoprecipitates with antibodies against the indicated proteins or normal IgG was probed with anti-ILEI antibody. ( f ) The crosslinked cell lysates were immunoprecipitated using normal IgG or anti-ILEI antibody. The blots were probed using the indicated antibodies. Full size image ILEI, which was originally identified in a database search for four-helix-bundle cytokines, is an evolutionarily conserved secretory protein [22] . ILEI is posttranslationally liberated from the membrane in secretory vesicles by cleavage of the signal sequence of the full-length (FL) precursor protein. Immunoblotting with an affinity-purified rabbit polyclonal anti-ILEI antibody revealed specific bands of 24 and 27 kDa in the conditioned medium and cell lysate of HEK293 cells, respectively, suggesting that the smaller species corresponded to a processed, secreted form of ILEI ( Fig. 1b ). Co-immunoprecipitation using native HEK293 cells indicated that antibodies against PS1, NCT, PEN-2 or APH-1 co-precipitated the precursor and processed forms of ILEI ( Fig. 1b ). The reverse assay revealed that the anti-ILEI antibody co-precipitated the four core components of the γ-secretase complex ( Fig. 1c ). Protein complex analysis using two-dimensional Blue Native SDS–PAGE suggested that ILEI is incorporated into multiple complexes of various molecular masses, one of which is comparable to that of the mature γ-secretase complex ( Fig. 1d ). These data confirmed the interaction between ILEI and the γ-secretase complex. To determine the partner that directly interacts with endogenous ILEI, we treated HEK293 cells in situ with a thiol-cleavable, membrane-permeable, chemical crosslinker. The cells were then lysed in a Nonidet P-40 buffer to dissociate non-crosslinked components of the γ-secretase complex. In this lysate, monomeric components of the γ-secretase complex were reduced by >80% on immunoblotting. PS1-CTF but not the other components co-immunoprecipitated ILEI ( Fig. 1e ). Conversely, the ILEI immunoprecipitates contained PS1-CTF but the other components were not present or were only faintly observed ( Fig. 1f ). These results suggest that ILEI directly binds to PS1-CTF. ILEI reduces Aβ generation by destabilizing APP-CTFβ RNA interference (RNAi)-mediated knockdown of endogenous ILEI in native HEK293 cells resulted in an approximately two-fold increase in Aβ40 and Aβ42 levels in the conditioned medium ( Fig. 2a ). Conversely, overexpression of ILEI decreased Aβ secretion ( Fig. 2b ). No significant alteration in the ratio of Aβ40 to Aβ42 was observed. ILEI knockdown or overexpression also increased or decreased APP intracellular domain generation, respectively ( Fig. 2c ). 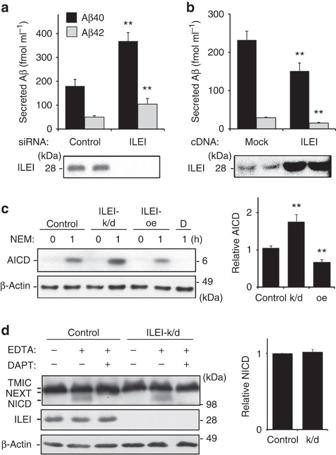Figure 2: ILEI inhibits cellular γ-secretase cleavage of APP but not Notch. Non-targeting control or ILEI-specific siRNA (a), or mock or ILEI cDNA (b) was transiently transfected into HEK293 cells. Aβ40 (black bars) and Aβ42 (grey bars) in the conditioned medium were measured using ELISA assays (n=6, mean±s.d.). **P<0.01 versus the control or the mock by Student’st-test. Lower panels show immunoblots of ILEI. (c) Immunoblot for APP intracellular domain (AICD) in control, ILEI-knockdown (k/d) or ILEI-overexpressing (oe) HEK293 cells. Cells were treated with 200 μMN-ethylmaleimide (NEM) for 1 h to block degradation of AICD60. AICD production was inhibited by DAPT (N-[N-(3,5-difluorophenacetyl)-L-alanyl]-S-phenylglycinet-butyl ester; 1 μM) treatment (d). The graph shows the relative intensity of AICD normalized to β-actin (n=3, mean±s.d.). **P<0.01 versus the control by Student’st-test. (d) Proteolysed derivatives of endogenous Notch-1 in control and ILEI-knockdown (k/d) mouse embryonic fibroblasts (MEFs). EDTA (1.5 mM) treatment induced cleavage of transmembrane/intracellular Notch (TMIC) to generate Notch extracellular truncation (NEXT), which was then cleaved by γ-secretase to release Notch intracellular domain (NICD). NICD production was inhibited by DAPT (1 μM) treatment. The graph shows the relative intensity of NICD normalized to β-actin (n=3, mean±s.d.). No significant difference versus the control was found (P>0.05 by Student’st-test). Figure 2: ILEI inhibits cellular γ-secretase cleavage of APP but not Notch. Non-targeting control or ILEI-specific siRNA ( a ), or mock or ILEI cDNA ( b ) was transiently transfected into HEK293 cells. Aβ40 (black bars) and Aβ42 (grey bars) in the conditioned medium were measured using ELISA assays ( n =6, mean±s.d.). ** P <0.01 versus the control or the mock by Student’s t -test. Lower panels show immunoblots of ILEI. ( c ) Immunoblot for APP intracellular domain (AICD) in control, ILEI-knockdown (k/d) or ILEI-overexpressing (oe) HEK293 cells. Cells were treated with 200 μM N -ethylmaleimide (NEM) for 1 h to block degradation of AICD [60] . AICD production was inhibited by DAPT ( N -[ N -(3,5-difluorophenacetyl)- L -alanyl]- S -phenylglycine t -butyl ester; 1 μM) treatment ( d ). The graph shows the relative intensity of AICD normalized to β-actin ( n =3, mean±s.d.). ** P <0.01 versus the control by Student’s t -test. ( d ) Proteolysed derivatives of endogenous Notch-1 in control and ILEI-knockdown (k/d) mouse embryonic fibroblasts (MEFs). EDTA (1.5 mM) treatment induced cleavage of transmembrane/intracellular Notch (TMIC) to generate Notch extracellular truncation (NEXT), which was then cleaved by γ-secretase to release Notch intracellular domain (NICD). NICD production was inhibited by DAPT (1 μM) treatment. The graph shows the relative intensity of NICD normalized to β-actin ( n =3, mean±s.d.). No significant difference versus the control was found ( P >0.05 by Student’s t -test). Full size image We next determined whether ILEI affects γ-secretase cleavage of the Notch-1 receptor. Treatment with EDTA enhances the site-2 cleavage of transmembrane/intracellular Notch to generate Notch extracellular truncation, which is then directly cleaved by γ-secretase to release Notch intracellular domain [23] . ILEI knockdown in mouse embryonic fibroblasts did not alter Notch intracellular domain generation from endogenous Notch in the presence of EDTA ( Fig. 2d ). In addition, we used a cell-based luciferase reporter assay for γ-secretase cleavage of Notch. The specificity was confirmed by treatment with a potent γ-secretase inhibitor, DAPT ( N -[ N -(3,5-difluorophenacetyl)- L -alanyl]- S -phenylglycine t -butyl ester), which attenuated luminescence (35.9±4.5% of vehicle; vehicle, 100.0±6.5%; n =5, P =0.000). Induction of luciferase activity was unaffected by transfection with ILEI siRNA (94.5±12.5% of control; control, 100.0±5.7%; n =5, P =0.449) or ILEI complementary DNA (96.8±8.9% of mock; mock, 100.0±8.2%; n =5, P =0.596). Thus, ILEI does not perturb γ-secretase processing of Notch. To test whether ILEI directly inhibits γ-secretase activity, we evaluated Aβ generation in a cell-free assay in which microsome fractions derived from HEK293 cells treated with non-targeting control or ILEI-specific siRNA were incubated with excess recombinant APP-CTFβ. Unexpectedly, we found no significant difference in Aβ generation ( n =6, P =0.851 for Aβ40; P =0.561 for Aβ42) between control (Aβ40: 3,253.3±399.0, Aβ42: 597.7±23.8 fmol ml −1 ) and ILEI-knockdown cells (Aβ40: 3,181.9±306.4, Aβ42: 614.5±28.9 fmol ml −1 ), indicating that ILEI reduces cellular Aβ generation without inhibiting γ-secretase activity. This result and the observation that ILEI was processed normally in the presence of DAPT ( Supplementary Fig. 2a ) further suggest that ILEI is not a competitive substrate of γ-secretase. In addition, ILEI knockdown did not detectably affect the cellular expression levels or subcellular localization of γ-secretase components, the intracellular trafficking of APP, or the Aβ secretion process ( Supplementary Figs 2b-d and 3a ). We also excluded the possibility that ILEI accelerated degradation of secreted Aβ in the culture medium ( Supplementary Fig. 3b ). Accordingly, ILEI knockdown increased the level of cellular APP-CTFs (APP-CTFα and APP-CTFβ) without augmenting APP-FL or secreted ectodomains of APP ( Fig. 3a ). ILEI knockdown did not change APP transcript expression as measured with quantitative real-time PCR (104.1±3.8% of control; control, 100.0±2.9%; n =3, P =0.291) or cellular β-secretase activity as measured with an in vitro assay (104.4±7.31% of control; control, 100.0±6.1%; n =3, P =0.555). We thus reasoned that ILEI knockdown stabilizes APP-CTFβ to increase Aβ generation. A cycloheximide chase assay indicated that ILEI knockdown significantly extended the half-life of APP-CTFs but not APP-FL ( Fig. 3b ). Altered ILEI expression levels did not change the levels of Beclin-1 or Rab5a or the subcellular localization of APP-CTFs ( Supplementary Fig. 3a and c ), suggesting that stabilization of APP-CTFs is not mediated by inactivation of general protein degradation through lysosomal/autophagosomal pathways or a defect in APP-CTF trafficking. The effect of ILEI knockdown on APP metabolism could be rescued by transfection of siRNA-resistant ILEI cDNA ( Fig. 3c ), ruling out potential off-target effects of the siRNA-mediated RNAi. 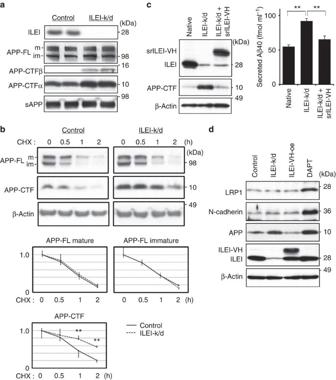Figure 3: ILEI knockdown selectively stabilizes APP-CTFs. (a) Immunoblots for APP and its proteolysed derivatives in control and ILEI-knockdown (k/d) HEK293 cells. The same amount of protein from cell lysates (for ILEI, APP FL and APP-CTFs) or conditioned medium (for secreted ectodomain; sAPP) was loaded. For APP-CTFβ, a longer exposure image is shown. m, mature; im, immature. (b) Immunoblots of APP-FL and APP-CTF in a cycloheximide (CHX) chase assay. m, mature; im, immature. Non-targeting control or ILEI-specific siRNA-transfected HEK293 cells were treated with 50 μg ml−1CHX for the indicated times. β-Actin was used as a loading control. The graphs below show the relative intensity of the bands (n=5, mean±s.d.). **P<0.01 versus the control by Student’st-test. (c) The restoring effect of siRNA-resistant ILEI-V5-His (srILEI-VH) on the levels of APP-CTFs and secreted Aβ. ILEI-specific siRNA-transfected HEK293 cells were further transfected with srILEI-VH. APP-CTF was analysed with immunoblotting, and secreted Aβ40 was measured with ELISA (n=3, mean±s.d.). **P<0.01 by Student’st-test. (d) Immunoblots for LRP1-CTF (25 kDa), N-cadherin-CTF (36 kDa) and APP-CTF (10 kDa) in control, stable ILEI-knockdown (k/d), stable ILEI-VH-overexpressing (oe) and DAPT (N-[N-(3,5-difluorophenacetyl)-L-alanyl]-S-phenylglycinet-butyl ester; 1 μM)-treated HEK293 cells. β-Actin was used as a loading control. Figure 3: ILEI knockdown selectively stabilizes APP-CTFs. ( a ) Immunoblots for APP and its proteolysed derivatives in control and ILEI-knockdown (k/d) HEK293 cells. The same amount of protein from cell lysates (for ILEI, APP FL and APP-CTFs) or conditioned medium (for secreted ectodomain; sAPP) was loaded. For APP-CTFβ, a longer exposure image is shown. m, mature; im, immature. ( b ) Immunoblots of APP-FL and APP-CTF in a cycloheximide (CHX) chase assay. m, mature; im, immature. Non-targeting control or ILEI-specific siRNA-transfected HEK293 cells were treated with 50 μg ml −1 CHX for the indicated times. β-Actin was used as a loading control. The graphs below show the relative intensity of the bands ( n =5, mean±s.d.). ** P <0.01 versus the control by Student’s t -test. ( c ) The restoring effect of siRNA-resistant ILEI-V5-His (srILEI-VH) on the levels of APP-CTFs and secreted Aβ. ILEI-specific siRNA-transfected HEK293 cells were further transfected with srILEI-VH. APP-CTF was analysed with immunoblotting, and secreted Aβ40 was measured with ELISA ( n =3, mean±s.d.). ** P <0.01 by Student’s t -test. ( d ) Immunoblots for LRP1-CTF (25 kDa), N-cadherin-CTF (36 kDa) and APP-CTF (10 kDa) in control, stable ILEI-knockdown (k/d), stable ILEI-VH-overexpressing (oe) and DAPT ( N -[ N -(3,5-difluorophenacetyl)- L -alanyl]- S -phenylglycine t -butyl ester; 1 μM)-treated HEK293 cells. β-Actin was used as a loading control. Full size image We examined whether ILEI also acts on low-density lipoprotein receptor-related protein 1 (LRP1) and N-cadherin, which are other substrates of γ-secretase. Knockdown or overexpression of ILEI did not affect accumulated levels of LRP1 or N-cadherin CTFs ( Fig. 3d ). Taken together with the results for Notch-1 ( Fig. 2d ), our results suggest that ILEI exhibits selectivity for APP-CTFs. ILEI interferes with the APP-CTF-stabilizing property of PS1 Processed ILEI is secreted from the cell, whereas intracellular ILEI is mostly associated with the microsome fraction ( Supplementary Fig. 4a ). Hence, we next determined whether extracellular application of a secreted form of ILEI decreased cellular Aβ secretion. We purified a recombinant polypeptide of processed ILEI from the conditioned medium of C-terminally V5-His-tagged ILEI (ILEI-VH)-overexpressing HEK293 cells ( Supplementary Fig. 4b ). When added into the culture medium of ILEI-knockdown HEK293 cells, purified ILEI-VH suppressed the levels of secreted Aβ and cellular APP-CTFs in a dose-dependent manner ( Fig. 4a ). Purified ILEI-VH was detected in perinuclear vesicular compartments and was associated with PS1 ( Fig. 4b,c ). These results suggest that ILEI acts on the extracellular side of the cell membrane and is endocytosed into the cell. In contrast, when we added purified ILEI-VH to cell-free mixtures and performed γ-secretase assays using microsome fractions derived from ILEI-knockdown HEK293 cells, Aβ generation was not altered ( Supplementary Fig. 4c ). 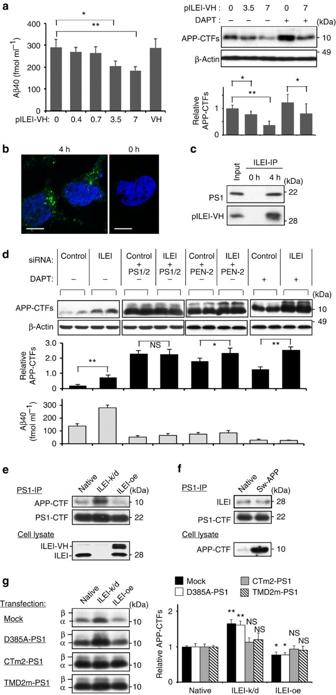Figure 4: Secreted ILEI interacts with the PS1/γ-secretase complex and interferes with its APP-CTF-stabilizing property. (a) Effects of purified ILEI-VH (pILEI-VH) on Aβ secretion and cellular APP-CTFs. pILEI-VH was added to the culture medium of ILEI-knockdown HEK293 cells at the indicated concentrations (μg ml−1). V5-His tag peptide (VH, 7 μg ml−1) served as a negative control. Secreted Aβ40 was measured with ELISA assay and APP-CTFs were analysed with immunoblotting. The right graph shows the relative intensity of APP-CTFs normalized to β-actin (n=3, mean±s.d.). (b) Laser scanning confocal microscopic images of pILEI-VH. pILEI-VH was immunostained with anti-V5 tag antibody (green) 0 or 4 h after its addition to the medium. Nuclei were stained with Hoechst 33342 (blue). Scale bar, 10 μm. (c) Co-immunoprecipitation assays for pILEI-VH and PS1. ILEI-knockdown HEK293 cells were lysed 0 or 4 h after addition of pILEI-VH, and the cell lysates were subjected to immunoprecipitation. A blot of the anti-ILEI precipitate was probed with anti-PS1-CTF or anti-V5 antibody. (d) ILEI-knockdown effects on APP-CTFs and secreted Aβ40 levels in PS1/PS2-knockdown, PEN-2-knockdown, or DAPT (N-[N-(3,5-difluorophenacetyl)-L-alanyl]-S-phenylglycinet-butyl ester; 1 μM)-treated HEK293 cells (n=3, mean±s.d.). (e) Co-immunoprecipitation assays for PS1 and APP-CTFs. Cell lysates of native, ILEI-knockdown (k/d) and ILEI-overexpressing (oe) HEK293 cells were immunoprecipitated with anti-PS1 antibody (PS1-IP). (f) Co-immunoprecipitation assays for PS1 and ILEI. Cell lysates of native and Swedish APP-overexpressing (Sw-APP) HEK293 cells were immunoprecipitated with anti-PS1 antibody (PS1-IP). (g) Effects of PS1 mutants on ILEI function. Mock, D385A-PS1, CTm2-PS1 or TMD2m-PS1 was transfected into native, ILEI-knockdown (k/d) and ILEI-overexpressing (oe) HEK293 cells (the same cell lines as ine). The same amount of protein from cell membrane lysates was subjected to immunoblotting for APP-CTFs. α: APP-CTFα, β: APP-CTFβ. The graph shows the relative intensity of APP-CTFs normalized to native HEK293 cells transfected with the same plasmid (n=3, mean±s.d.). For data froma,dandg, two-tailed Student’st-test was used to analyse statistical significance. *P<0.05, **P<0.01 and NS, not significant, versus control (a,d) or native (g). Figure 4: Secreted ILEI interacts with the PS1/γ-secretase complex and interferes with its APP-CTF-stabilizing property. ( a ) Effects of purified ILEI-VH (pILEI-VH) on Aβ secretion and cellular APP-CTFs. pILEI-VH was added to the culture medium of ILEI-knockdown HEK293 cells at the indicated concentrations (μg ml −1 ). V5-His tag peptide (VH, 7 μg ml −1 ) served as a negative control. Secreted Aβ40 was measured with ELISA assay and APP-CTFs were analysed with immunoblotting. The right graph shows the relative intensity of APP-CTFs normalized to β-actin ( n =3, mean±s.d.). ( b ) Laser scanning confocal microscopic images of pILEI-VH. pILEI-VH was immunostained with anti-V5 tag antibody (green) 0 or 4 h after its addition to the medium. Nuclei were stained with Hoechst 33342 (blue). Scale bar, 10 μm. ( c ) Co-immunoprecipitation assays for pILEI-VH and PS1. ILEI-knockdown HEK293 cells were lysed 0 or 4 h after addition of pILEI-VH, and the cell lysates were subjected to immunoprecipitation. A blot of the anti-ILEI precipitate was probed with anti-PS1-CTF or anti-V5 antibody. ( d ) ILEI-knockdown effects on APP-CTFs and secreted Aβ40 levels in PS1/PS2-knockdown, PEN-2-knockdown, or DAPT ( N -[ N -(3,5-difluorophenacetyl)- L -alanyl]- S -phenylglycine t -butyl ester; 1 μM)-treated HEK293 cells ( n =3, mean±s.d.). ( e ) Co-immunoprecipitation assays for PS1 and APP-CTFs. Cell lysates of native, ILEI-knockdown (k/d) and ILEI-overexpressing (oe) HEK293 cells were immunoprecipitated with anti-PS1 antibody (PS1-IP). ( f ) Co-immunoprecipitation assays for PS1 and ILEI. Cell lysates of native and Swedish APP-overexpressing (Sw-APP) HEK293 cells were immunoprecipitated with anti-PS1 antibody (PS1-IP). ( g ) Effects of PS1 mutants on ILEI function. Mock, D385A-PS1, CTm2-PS1 or TMD2m-PS1 was transfected into native, ILEI-knockdown (k/d) and ILEI-overexpressing (oe) HEK293 cells (the same cell lines as in e ). The same amount of protein from cell membrane lysates was subjected to immunoblotting for APP-CTFs. α: APP-CTFα, β: APP-CTFβ. The graph shows the relative intensity of APP-CTFs normalized to native HEK293 cells transfected with the same plasmid ( n =3, mean±s.d.). For data from a , d and g , two-tailed Student’s t -test was used to analyse statistical significance. * P <0.05, ** P <0.01 and NS, not significant, versus control ( a , d ) or native ( g ). Full size image Although we identified ILEI as a γ-secretase complex-binding protein, whether ILEI interaction with the γ-secretase complex mediated the stabilization of APP-CTFs was not clear. To address this issue, we tested the effect of ILEI knockdown on APP-CTF levels in PS1/PS2-knockdown HEK293 cells. High levels of APP-CTFs accumulated in PS1/PS2-knockdown cells in which the γ-secretase complex was ablated. ILEI knockdown did not lead to any further increase in APP-CTFs ( Fig. 4d ). In contrast, as shown in Fig. 4d , the APP-CTF level was increased by ILEI knockdown in PEN-2-knockdown HEK293 cells, which exclusively contained immature, inactive γ-secretase complexes [24] . Furthermore, ILEI knockdown and ILEI-VH treatment enhanced and reduced accumulation of APP-CTFs in the presence of a γ-secretase inhibitor, respectively ( Fig. 4a,d ). Thus, ILEI requires interaction with the γ-secretase complex, regardless of whether the complex is enzymatically active or inactive, to alter the stability of APP-CTFs. In contrast, co-immunoprecipitation assays revealed no direct interaction between ILEI and APP-CTFs ( Supplementary Fig. 3d ). We next asked whether ILEI competes with APP-CTFs for binding with the γ-secretase complex. Co-immunoprecipitation assays indicated that the amount of PS1-bound APP-CTFs was inversely correlated with the ILEI expression level ( Fig. 4e ). In contrast, alternative co-immunoprecipitation assays suggested that the expression level of APP did not influence the amount of PS1-bound ILEI ( Fig. 4f ). These results imply that ILEI non-competitively interferes with the binding between the γ-secretase complex and APP-CTFs. The PS1/γ-secretase complex stably binds APP-CTFs and protects them from non-specific degradation [21] , [25] . Analysis of the APP-CTF-stabilizing property is hampered by γ-secretase activity, although the former is independent of the latter [25] . To determine whether ILEI interferes with this property, we used three catalytically inactive PS1 mutants: D385A-PS1, CTm2-PS1 and TMD2m-PS1. D385A-PS1 has an alanine substitution of the aspartic acid residue (D 385 ) at the active centre and binds with APP-CTFs and ILEI ( Supplementary Fig. 5a–c ). CTm2-PS1 has alanine substitutions of D 385 and the sequential three amino acid residues (D 458 , Q 459 and L 460 ) in the extracellular/luminal C-terminal tail and lacks the ability to bind ILEI ( Supplementary Fig. 5a,b ). TMD2m-PS1, the second transmembrane domain (TMD) of which is replaced with the TMD of CD4 (ref. 26 ), lacks the ability to bind APP-CTFs ( Supplementary Fig. 5c ). Overexpression of D385A-PS1 or CTm2-PS1 but not TMD2m-PS1 increased APP-CTFs in PS1/PS2-double knockout mouse embryonic fibroblasts [27] ( Supplementary Fig. 5d ), suggesting that APP-CTFs are stabilized by the binding with PS1. The APP-CTF-destabilizing effect of ILEI was abrogated by overexpression of CTm2-PS1 or TMD2m-PS1 ( Fig. 4g ), suggesting that both mutants prevented ILEI from destabilizing APP-CTFs in a dominant-negative manner. Exogenous CTm2-PS1 and TMD2m-PS1 are expected to compete with endogenous PS1 for binding to APP-CTFs and ILEI, respectively. Our results thus imply that APP-CTF destabilization by ILEI requires the interaction between ILEI and PS1, and between PS1 and APP-CTFs. APP-CTFs that accumulated with ILEI knockdown were indeed colocalized with PS1 in subcellular fractions of cultured cells ( Supplementary Fig. 3a ). These results support our hypothesis that ILEI binds to the PS1/γ-secretase complex and interferes with its APP-CTF-stabilizing property to reduce Aβ generation. Neuronal expression of ILEI Previous studies showed that ILEI is expressed in the central nervous system as well as in secretory epithelia [22] , [28] . However, the regional and cellular distribution of ILEI in mammalian brains has not been examined. We confirmed the specificity of rabbit anti-ILEI antibody ( Supplementary Fig. 6 ) and performed immunohistochemical staining for ILEI. ILEI was widely expressed in mouse and human brains, and was prominent in pyramidal neurons in the cerebral cortex and hippocampus. ILEI-immunoreactive structures were detected in perinuclear regions of neuronal cell bodies, whereas glial fibrillary acidic protein-positive astrocytes and Iba1-positive microglia were negative for ILEI ( Fig. 5a ). Perinuclear ILEI was colocalized with TGN46, Rab5a and Rab7, indicating that ILEI principally resides in the trans -Golgi network and the endocytic vesicles where Aβ is reportedly produced [29] , [30] ( Supplementary Fig. 7 ). Colocalization of ILEI and APP-CTFs was also confirmed ( Supplementary Fig. 8 ). 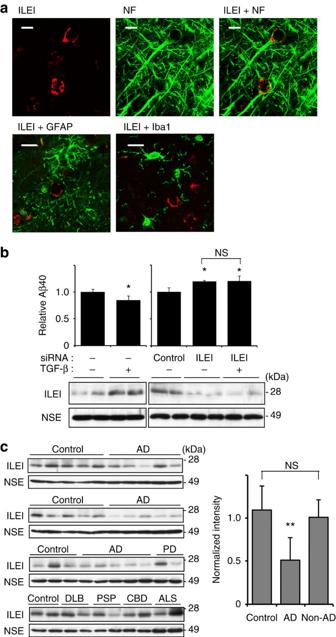Figure 5: Neuronal expression of ILEI is induced by TGF-β and reduced in AD brains. (a) Double immunostaining for ILEI and cell type-specific markers in mouse brain sections. Neurofilament (NF), glial fibrillary acidic protein (GFAP) and Iba-I are marker proteins for neurons, astrocytes and microglia, respectively. Scale bars, 10 μm. (b) Effects of TGF-β treatment on cultured rat brain slices pretreated with non-targeting control or ILEI-specific siRNA. Forebrain slices containing the hippocampus and cerebral cortex were prepared from three Wistar rats (3-week-old, female). The relative levels of Aβ40 (n=3, mean±s.d.) and immunoblotting for ILEI are shown. Neuron-specific enolase (NSE) was used as a loading control. *P<0.05 versus vehicle or control, and NS, not significant by Student’st-test. Aβ40 concentrations were as follows: control for TGF-β, 743.68±39.32; TGF-β, 631.23±54.36; control for ILEI-knockdown, 751.77±60.23; ILEI-knockdown, 901.28±12.61; ILEI-knockdown/TGF-β, 902.28±72.57 pmol per g protein (n=3, mean±s.d.). (c) Immunoblots for ILEI in Tris-buffered saline-extracted fractions from temporal cortices of AD patients (n=15, 82.0±4.5 years old, post-mortem interval 7.0±3.5 h), age-matched controls without neurological disease (n=15, 80.1±1.7 years old, post-mortem interval 8.0±5.4 h) and non-AD neurological disease controls (n=10, 79.6±3.7 years old, post-mortem interval 9.3±5.9 h). Non-AD disease controls were Parkinson’s disease (PD), dementia with Lewy bodies (DLB), progressive supranuclear palsy (PSP), corticobasal degeneration (CBD) or amyotrophic lateral sclerosis (ALS). The graph shows the relative intensity of ILEI normalized to NSE (mean±s.d.). **P<0.01 versus control or non-AD control and NS, not significant by Student’st-test. Figure 5: Neuronal expression of ILEI is induced by TGF-β and reduced in AD brains. ( a ) Double immunostaining for ILEI and cell type-specific markers in mouse brain sections. Neurofilament (NF), glial fibrillary acidic protein (GFAP) and Iba-I are marker proteins for neurons, astrocytes and microglia, respectively. Scale bars, 10 μm. ( b ) Effects of TGF-β treatment on cultured rat brain slices pretreated with non-targeting control or ILEI-specific siRNA. Forebrain slices containing the hippocampus and cerebral cortex were prepared from three Wistar rats (3-week-old, female). The relative levels of Aβ40 ( n =3, mean±s.d.) and immunoblotting for ILEI are shown. Neuron-specific enolase (NSE) was used as a loading control. * P <0.05 versus vehicle or control, and NS, not significant by Student’s t -test. Aβ40 concentrations were as follows: control for TGF-β, 743.68±39.32; TGF-β, 631.23±54.36; control for ILEI-knockdown, 751.77±60.23; ILEI-knockdown, 901.28±12.61; ILEI-knockdown/TGF-β, 902.28±72.57 pmol per g protein ( n =3, mean±s.d.). ( c ) Immunoblots for ILEI in Tris-buffered saline-extracted fractions from temporal cortices of AD patients ( n =15, 82.0±4.5 years old, post-mortem interval 7.0±3.5 h), age-matched controls without neurological disease ( n =15, 80.1±1.7 years old, post-mortem interval 8.0±5.4 h) and non-AD neurological disease controls ( n =10, 79.6±3.7 years old, post-mortem interval 9.3±5.9 h). Non-AD disease controls were Parkinson’s disease (PD), dementia with Lewy bodies (DLB), progressive supranuclear palsy (PSP), corticobasal degeneration (CBD) or amyotrophic lateral sclerosis (ALS). The graph shows the relative intensity of ILEI normalized to NSE (mean±s.d.). ** P <0.01 versus control or non-AD control and NS, not significant by Student’s t -test. Full size image Recently, transforming growth factor-β (TGF-β) signalling in neuronal cells was reported to lead to decreased levels of APP-CTF and Aβ [31] . On the other hand, TGF-β selectively induces translation of ILEI via phosphorylation of heterogeneous nuclear ribonucleoprotein E1 in mammary gland cells [32] . Thus, we asked whether the inhibitory effect of TGF-β on Aβ production in brain is mediated by ILEI induction. To address this, we first examined ILEI induction and Aβ reduction by TGF-β using organotypic culture of rat forebrain slices. Next, we evaluated TGF-β-induced reduction in Aβ production from forebrain slices pretreated with ILEI-specific siRNA. TGF-β induced ILEI and reduced Aβ secretion, and these effects were almost completely abrogated in the ILEI-knockdown condition ( Fig. 5b ). To evaluate the possible involvement of ILEI in AD pathogenesis, we examined the levels of secreted ILEI in autopsy brains of patients with sporadic AD. Soluble fractions from temporal cortex homogenates were subjected to immunoblotting. ILEI expression was normalized to the level of neuron-specific enolase in each sample to compensate for the difference in neuronal density. ILEI was significantly reduced in AD cases compared with age-matched non-neurological disease controls ( Fig. 5c , P =0.000) and was inversely correlated with levels of Aβ or phosphorylated tau with semi-quantitative immunoblotting ( Supplementary Fig. 9a,b ). The ILEI level in autopsy brains with non-AD neurological diseases was equivalent to that of non-neurological disease control brains ( Fig. 5c , P =0.459). Although our result is preliminary due to the limited number of cases examined, the trend is unequivocal. The decrease in ILEI did not seem to be secondary to brain Aβ accumulation, because ILEI is unaltered in the brains of aged APP-overexpressing mice [33] ( Supplementary Fig. 9c ). ILEI ameliorates the phenotypes of AD model mice To analyse the consequences of ILEI overexpression in mammalian brains, we developed Tg mice in which the mouse prion promoter was used to drive expression of a human ILEI cDNA transgene predominantly in the brain [34] . Heterozygous Tg mice exhibited normal development and fertility with no gross morphological defects. Similar to wild-type mice, ILEI expression was restricted to neuronal cells in the brains of Tg mice ( Fig. 6a ). Immunoblotting of brain homogenates indicated a three-fold increase in ILEI protein levels and no alteration in Notch intracellular domain levels in the Tg mice compared with non-Tg littermates ( Fig. 6b ). These findings suggest that the ILEI-Tg mice represent an appropriate model for ILEI overexpression without obvious ectopic expression. Immunoblotting revealed a 30% decrease in APP-CTFα and APP-CTFβ levels in the brains of Tg mice compared with controls ( Fig. 6c ), and the endogenous levels of Aβ40 and Aβ42 in Tris-buffered saline-soluble and -insoluble fractions of brain homogenates were significantly reduced in ILEI-Tg mice compared with non-Tg littermate controls ( Fig. 6d ). Thus, overexpression of ILEI suppresses APP-CTF accumulation and Aβ generation in vivo while sparing Notch processing. 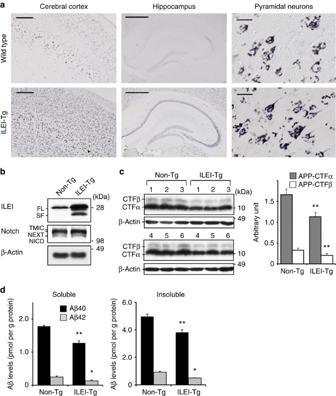Figure 6: The Aβ level is reduced in brains of ILEI-Tg mice. (a) Immunostaining shows ILEI expression in neurons of the cerebral cortex and hippocampus of wild-type and ILEI-Tg mouse brains (8 months old). Scale bars, 200 μm (left), 500 μm (centre), 20 μm (right). (b) Immunoblots for ILEI and Notch in brains of ILEI-Tg mice and non-Tg littermates (6 months old). β-Actin was used as a loading control. FL, full-length; SF, secreted form. (c) Immunoblots for APP-CTFs in brains of ILEI-Tg mice and non-Tg littermates (6–8 months old,n=6 per genotype). The graph shows the relative intensity of APP-CTFs normalized to β-actin (n=6, mean±s.d.). **P<0.01 versus non-Tg mice by Student’st-test. (d) Brain Aβ levels in non-Tg and ILEI-Tg mice (10 months old,n=6 per genotype). Aβ40 (black bars) and Aβ42 (grey bars) in Tris-buffered saline-soluble and -insoluble fractions of brain homogenates were measured using ELISA assays (n=6, mean±s.d.). *P<0.05 and **P<0.01 versus non-Tg by Student’st-test. Figure 6: The Aβ level is reduced in brains of ILEI-Tg mice. ( a ) Immunostaining shows ILEI expression in neurons of the cerebral cortex and hippocampus of wild-type and ILEI-Tg mouse brains (8 months old). Scale bars, 200 μm (left), 500 μm (centre), 20 μm (right). ( b ) Immunoblots for ILEI and Notch in brains of ILEI-Tg mice and non-Tg littermates (6 months old). β-Actin was used as a loading control. FL, full-length; SF, secreted form. ( c ) Immunoblots for APP-CTFs in brains of ILEI-Tg mice and non-Tg littermates (6–8 months old, n =6 per genotype). The graph shows the relative intensity of APP-CTFs normalized to β-actin ( n =6, mean±s.d.). ** P <0.01 versus non-Tg mice by Student’s t -test. ( d ) Brain Aβ levels in non-Tg and ILEI-Tg mice (10 months old, n =6 per genotype). Aβ40 (black bars) and Aβ42 (grey bars) in Tris-buffered saline-soluble and -insoluble fractions of brain homogenates were measured using ELISA assays ( n =6, mean±s.d.). * P <0.05 and ** P <0.01 versus non-Tg by Student’s t -test. Full size image To determine whether ILEI overexpression affects disease progression, we bred ILEI-Tg mice with Swedish mutant APP-overexpressing mice (APP-Tg, Tg2576), which show impaired learning and memory and brain Aβ deposition by 9–10 months of age [33] . APP/ILEI-double Tg mice appeared healthy and had a survival curve comparable with APP-Tg mice. We used a Y-maze test to assess hippocampus-dependent spatial working memory, which declines with age in APP-Tg mice [33] . At 11–13 months of age, but not at 6 months of age, APP-Tg mice showed poor performance ( n =12, P =0.0000), but APP/ILEI-Tg mice showed similar performance ( n =11, P =0.3692) compared with non-Tg littermate ( Fig. 7a ). We found no significant difference in locomotor activity or motivation to explore the maze (the total number of arm entries was 28.6±3.75 in APP-Tg mice and 25.2±4.08 in APP/ILEI-Tg mice; P =0.5478). 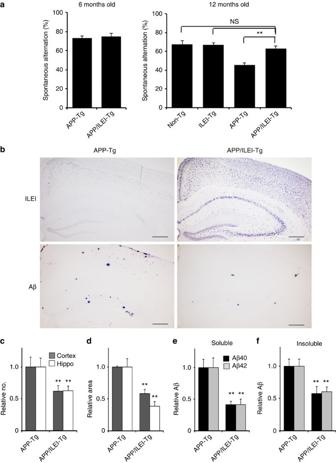Figure 7: ILEI overexpression ameliorates the memory deficit and reduces brain Aβ burden in APP-Tg mice. (a) Spontaneous alternation in the Y-maze test. APP-Tg (3 females at 6 months age, 6 males and 6 females at 12 months age), ILEI-Tg (5 males and 4 females at 12 months age), APP/ILEI-Tg (3 females at 6 months age, 5 males and 6 females at 12 months age) and non-Tg (5 males and 4 females at 12 months age) littermate mice were used. Data are expressed as percentage (mean±s.e.m.). **P<0.01, NS, not significant by Student’st-test. (b) Immunostaining images with anti-ILEI antibody (top) and anti-Aβ antibody (bottom) using serial brain sections from 12-month-old APP-Tg (left) and APP/ILEI-Tg (right) mice. Scale bars, 200 μm. (c–f) Aβ burden in brains of APP-Tg and APP/ILEI-Tg mice (12 months old,n=6 per genotype). The plaque number (c) and the area occupied by plaques (d) in Aβ-immunostained sections of prefrontal cortex (grey bars) and hippocampus (white bars) (mean±s.e.m.). The relative levels of Aβ40 (black bars) and Aβ42 (grey bars) in soluble (e) and insoluble (f) fractions (mean±s.e.m.). **P<0.01 versus the APP-Tg by Student’st-test. Aβ concentrations were as follows: soluble Aβ40 of APP-Tg, 19.79±2.66; soluble Aβ42 of APP-Tg, 4.69±0.72; insoluble Aβ40 of APP-Tg, 1362.56±152.88; insoluble Aβ42 of APP-Tg, 517.80±57.82; soluble Aβ40 of APP/ILEI-Tg, 8.14±1.21; soluble Aβ42 of APP/ILEI-Tg, 1.95±0.42; insoluble Aβ40 of APP/ILEI-Tg, 788.68±142.23; insoluble Aβ42 of APP/ILEI-Tg, 312.92±38.80 pmol per g protein (mean±s.e.m.). Figure 7: ILEI overexpression ameliorates the memory deficit and reduces brain Aβ burden in APP-Tg mice. ( a ) Spontaneous alternation in the Y-maze test. APP-Tg (3 females at 6 months age, 6 males and 6 females at 12 months age), ILEI-Tg (5 males and 4 females at 12 months age), APP/ILEI-Tg (3 females at 6 months age, 5 males and 6 females at 12 months age) and non-Tg (5 males and 4 females at 12 months age) littermate mice were used. Data are expressed as percentage (mean±s.e.m.). ** P <0.01, NS, not significant by Student’s t -test. ( b ) Immunostaining images with anti-ILEI antibody (top) and anti-Aβ antibody (bottom) using serial brain sections from 12-month-old APP-Tg (left) and APP/ILEI-Tg (right) mice. Scale bars, 200 μm. ( c – f ) Aβ burden in brains of APP-Tg and APP/ILEI-Tg mice (12 months old, n =6 per genotype). The plaque number ( c ) and the area occupied by plaques ( d ) in Aβ-immunostained sections of prefrontal cortex (grey bars) and hippocampus (white bars) (mean±s.e.m.). The relative levels of Aβ40 (black bars) and Aβ42 (grey bars) in soluble ( e ) and insoluble ( f ) fractions (mean±s.e.m.). ** P <0.01 versus the APP-Tg by Student’s t -test. Aβ concentrations were as follows: soluble Aβ40 of APP-Tg, 19.79±2.66; soluble Aβ42 of APP-Tg, 4.69±0.72; insoluble Aβ40 of APP-Tg, 1362.56±152.88; insoluble Aβ42 of APP-Tg, 517.80±57.82; soluble Aβ40 of APP/ILEI-Tg, 8.14±1.21; soluble Aβ42 of APP/ILEI-Tg, 1.95±0.42; insoluble Aβ40 of APP/ILEI-Tg, 788.68±142.23; insoluble Aβ42 of APP/ILEI-Tg, 312.92±38.80 pmol per g protein (mean±s.e.m.). Full size image We next quantified the Aβ plaque load using brain sections immunohistochemically stained for Aβ. At 12 months of age, the plaque number and the area occupied by plaques in the cerebral cortex and hippocampus were clearly reduced in APP/ILEI-Tg mice compared with APP-Tg littermates ( Fig. 7b–d ). Moreover, quantitative analysis with Aβ enzyme-linked immunosorbent assay (ELISA) using brains of the same set of mice confirmed that the levels of Aβ40 and Aβ42 in soluble and insoluble fractions were significantly lower in APP/ILEI-Tg mice than in APP-Tg littermates ( Fig. 7e,f ). These results support the conclusion that ILEI efficiently reduces Aβ accumulation and ameliorates the memory deficit caused by Aβ overload in the brain. Our study shows that Aβ generation can be attenuated by overexpression or administration of ILEI. ILEI regulated Aβ generation by altering the stability of APP-CTFs by extracellular or luminal binding to the PS1/γ-secretase complex. ILEI exhibited functional selectivity for APP and did not affect Notch derivatives. Neuronal expression of ILEI was enhanced by TGF-β signalling in mammalian brain. The levels of secreted ILEI were reduced in autopsy brains of patients with sporadic AD. Tg overexpression of ILEI successfully ameliorated brain Aβ burden and memory deficits in AD model mice. Based on a recent structural study showing that ILEI and pancreatic-derived factor (PANDER, also known as FAM3B) adopt a globular ββα fold that is distinct from the conformation of classical cytokines, the FAM3 superfamily members may represent a novel class of signalling molecules [35] . Earlier works have revealed that ILEI acts downstream of TGF-β to induce epithelial-to-mesenchymal transition of epithelial cells, whereas PANDER, which is cosecreted with insulin from pancreatic islet cells, is involved in regulation of insulin secretion and glycemic levels [28] , [36] , [37] . Expression of the ILEI transcript in human brain has been described [22] . However, the function of ILEI in the nervous system remains largely unknown, except for its possible role in development of the Xenopus retina [38] . Our results suggest that ILEI is induced by TGF-β also in mammalian brain. Multiple lines of evidence link TGF-β signalling to brain Aβ accumulation and development of AD [39] . Thus, the specific genotype +10 C/C of the TGF-β1 gene, which affects the expression level of TGF-β1, is associated with an increased risk of AD [40] , and the neuronal expression of TGF-β type II receptors is reduced in AD brains from the early stage of disease development [31] . In addition, recent proteomic analysis of cerebrospinal fluid revealed significantly decreased ILEI levels in patients with idiopathic temporal lobe epilepsy [41] , in whom the age-related incidence of Aβ plaques in temporal cortex is significantly higher compared with age-matched controls [42] . The ILEI level in cerebrospinal fluid may also be a biomarker for AD [43] . These reports indirectly support our conclusion, indicating the functional relevance of ILEI to Aβ generation in vivo and the pathogenesis of AD. A previous study using cultured neurons derived from APP-CTFβ-Tg mice indicated that 30% of APP-CTFβ is converted to Aβ [44] . APP-CTFs are also degraded through alternative pathways, including proteasomal, lysosomal and autophagosomal-lysosomal pathways [44] , [45] , [46] , [47] . In cultured neuronal cells, proteasome inhibition increases Aβ generation by augmenting the amount of APP-CTFβ [44] , [45] . Hence, ILEI knockdown may increase Aβ generation by inhibiting APP-CTFβ degradation through pathways that do not lead to Aβ production. Alteration of APP-CTF stability by ILEI required cellular expression of the γ-secretase complex, regardless of whether the complex was enzymatically active or inactive. A large pool of the PS1/γ-secretase complexes remains catalytically inactive in the cell [48] . Even active γ-secretase complexes stably bind to APP-CTFs on substrate-docking sites, which are spatially separated from the catalytic centre [21] , [49] . Enhanced expression of PS1 in cultured insect and mammalian cells increases the accumulated level of APP-CTFβ by extending its half-life independent of γ-secretase activity [25] . Thus, the PS1/γ-secretase complex also functions as a chaperone that protects APP-CTFs from nonspecific degradation. Chaperone properties of the γ-secretase complex have been described only for APP but not for other substrates. Our results indicate that ILEI inhibits this stabilizing ability by directly binding to PS1-CTF without inhibiting γ-secretase activity, resulting in decreased accumulation of APP-CTFs and diminished generation of Aβ. This possibility is supported by the finding that ILEI is localized in the trans -Golgi network and the endocytic vesicles where PS1:CTFβ complexes are located and Aβ is produced [29] , [30] . Several proteins regulate the stability of APP by directly binding or phosphorylating its cytoplasmic domain [50] . In contrast, ILEI selectively accelerated γ-secretase-independent degradation of APP-CTFs through a novel mechanism in which ILEI interacted with the PS1/γ-secretase complex but not APP on the extracellular or luminal side of the membrane. Modifier of cell adhesion, which is known as dedicator of cytokinesis 3, a member of the dedicator of cytokinesis family of guanine nucleotide exchange factors, binds presenilins and selectively accelerates proteasome-mediated degradation of APP [51] . However, in contrast to ILEI, modifier of cell adhesion is a cytoplasmic protein that binds to presenilins on the cytoplasmic side of the membrane and destabilizes both APP-FL and APP-CTFs via an unknown mechanism [52] . Conversely, platelet-activating factor acetylhydrolase, isoform 1b, subunit 2 and sphingolipids inhibit γ-secretase-independent degradation of APP-CTFs and increase Aβ production [53] , [54] . Previous studies have revealed a significant increase in APP-CTFβ as well as Aβ in sporadic AD brains, which is sometimes associated with hyperactivity of β-secretase/BACE1 or downregulation of TGF-β signalling [5] , [6] , [31] . In addition, the protein degradation activities of proteasomes, lysosomes and autophagy gradually decline with age and contribute to high levels of APP-CTFβ and Aβ, and consequently to an increased risk of sporadic AD [7] , [8] , [45] . On the other hand, clinical trials using non-selective inhibitors of γ-secretase activity were discontinued due to adverse effects that were probably caused by Notch inhibition and APP-CTF accumulation [11] , [12] , [13] , [55] . Thus, ILEI may be a plausible target for the development of disease-modifying therapies for AD, because ILEI may alter disease progression without perturbing Notch signalling and increasing APP-CTFβ. Plasmids For construction of srPEN-2 (ref. 24 ), three silent nucleotide substitutions were introduced into human PEN-2 cDNA by PCR-based site-directed mutagenesis using the primer: 5′-GAACAGAGCCAAATCAAAGGTTACGTATGGCGCTCAGCTGTGGGCTTCCTCTTC-3′. The pcDNA3-TAP plasmid containing DNA for the TAP tag, which consists of two immunoglobulin-binding domains of protein A from Staphylococcus aureus , a cleavage site for the tobacco etch virus (TEV) protease and the calmodulin-binding polypeptide, was obtained from Dr K. Oshikawa (Kyushu Universiy, Fukuoka, Japan). To generate pTAP-srPEN-2, the TAP tag fragment was fused in-frame to the 5′-end of srPEN-2 cDNA in pcDNA4 (Invitrogen, Carlsbad, CA, USA). A cDNA encoding ILEI with or without the stop codon was amplified from a human brain cDNA library (Clontech, San Diego, CA, USA) using PCR and was then ligated into pcDNA6/V5-His (Invitrogen). To construct the ILEI knockdown vector, the oligonucleotide 5′-GGAGAAGUAUUAGACACU-3′ was ligated into pSUP (Oligoengine, Seattle, WA, USA). To prepare an expression plasmid for siRNA-resistant ILEI, five neutral mutations were introduced into ILEI cDNA by PCR-based site-directed mutagenesis using the primer: 5′-GAAAAACAGGAGAGGTTCTGGATACTAAATATTTTG-3′. The expression plasmids for PS1 mutants were constructed by PCR-based mutagenesis using the expression plasmid for wild-type human PS1 (ref. 56 ) as template. The sequences of all constructs were confirmed by sequencing. NotchΔE [57] and HES-Y [58] are gifts from Drs Raphael Kopan (Washington University, St Louis, MO, USA) and Masayasu Okochi (Osaka University, Osaka, Japan), respectively. Identification of ILEI To generate the HEK-TAP-PEN-2 and HEK-TAP empty cell lines, we transfected HEK293 cells (CRL-1573, ATCC) stably expressing PEN-2-specific siRNA with pTAP-srPEN-2 or pTAP-empty. HEK-TAP-PEN-2 or HEK-TAP-empty cells were homogenized in buffer A (20 mM Tris (pH 7.5), 150 mM NaCl, 0.5 mM EDTA) containing a protease inhibitor cocktail (Roche Diagnostics, Mannheim, Germany). The postnuclear supernatants were centrifuged at 100,000 g for 1 h to collect the microsome membrane pellets. The pellet was solubilized in buffer A containing 1% CHAPSO and then mixed with IgG-sepharose beads followed by incubation at 4 °C for 2 h. The mixture was washed with buffer A containing 0.5% CHAPSO. The beads were incubated with 10 U of TEV protease in TEV buffer (10 mM Tris (pH 8.0), 150 mM NaCl, 0.5 mM EDTA, 0.5% CHAPSO) at 4 °C for 12 h. After adjustment of the calcium concentration to 200 μM, the supernatant was mixed with calmodulin resin in three volumes of buffer B (10 mM Tris (pH 8.0), 150 mM NaCl, 1 mM Mg acetate, 1 mM imidazol, 2 mM CaCl 2 , 0.5% CHAPSO) and then incubated for 5 h at 4 °C. The proteins were eluted with SDS sample buffer and subjected to SDS–PAGE. The gel was stained with silver or SYPRO Ruby (Molecular Probes, Eugene, OR, USA). Bands were excised from the gel, and proteins in each gel piece that contained a specific band or a group of specific bands were digested with trypsin and subjected to liquid chromatography-tandem mass spectrometry followed by a search of the Mascot database. Immunoblotting analysis The same amount of protein from cell lysates was loaded onto SDS–PAGE and transferred to a polyvinylidene fluoride membrane (Millipore, Billerica, MA, USA) or nitrocellurose membrane (BioRad, Hercules, CA, USA). The membranes were incubated with the following primary antibodies at 4 °C overnight, washed and incubated with corresponding horseradish peroxidase-conjugated secondary antibodies (1:3,500, Invitrogen) for 1 h. Anti-human ILEI polyclonal antibody was raised in rabbits against a thyroglobulin-conjugated synthetic polypeptide corresponding to amino acid residues 126 to 143 with an added amino-terminal Cys residue (C+GGDVAPFIEFLKAIQDGT). This antibody was purified using immunoaffinity chromatography with immobilized antigen (1:4,000). The following antibodies were also used: goat polyclonal anti-FAM3C antibody (1:2,000, R&D Systems, Minneapolis, MN, USA); rabbit polyclonal anti-NCT (1:5,000), anti-APP-CTF (1:10,000) and mouse monoclonal anti-β-actin (1:10,000) antibodies (Sigma, St Louis, MO, USA); mouse monoclonal anti-PS1 loop antibody (1:3,500, Chemicon, Temecula, CA, USA); rabbit polyclonal anti-APH-1L antibody (1:2,000, Covance, Princeton, NJ, USA); rabbit polyclonal anti-PEN-2 antibody (1:2,000, Calbiochem, San Diego, CA, USA); mouse monoclonal anti-Notch-1 antibody (mN1A, 1:1,000, AbD Serotec, Kidlington, UK); rabbit monoclonal anti-LRP1 antibody (1:5,000, Abcam, Cambridge, MA, USA); rabbit polyclonal anti-cadherin antibody (1:10,000, Sigma); mouse monoclonal antibody specific for the 17–26 amino acid residues of the human Aβ (4G8, 1:1,000, Covance); rabbit polyclonal anti-neuron-specific enolase (1:10,000, Assay Biotechnology, Sunnyvale, CA, USA). Original immunoblots can be found in Supplementary Fig. 10 . Co-immunoprecipitation and chemical crosslinking Cultured cells were lysed in a lysis buffer containing 1% CHAPSO. After pre-clearing with protein G-Sepharose 4 fast flow (GE Healthcare, Tokyo, Japan) for 1 h, postnuclear supernatants were incubated with the appropriate antibody. The immunoprecipitates were recovered by overnight incubation with protein G-Sepharose and were analysed with immunoblotting. To eliminate IgG light-chain bands on immunoblots, signals were detected with horseradish peroxidase-conjugated bio-nanocapsules incorporating IgG Fc-binding Z domains derived from S. aureus protein A [59] (Beacle, Kyoto, Japan) instead of the secondary antibody. For crosslinking, HEK293 cells were treated with 2 mM dithiobis succinimidyl propionate (Thermo Fisher Scientific, Kanagawa, Japan) for 2 h on ice. The reaction was stopped by adding Tris–HCl (pH 7.5, final 20 mM). After incubating on ice for 15 min, the cells were lysed with a lysis buffer containing 1% Nonidet P-40. Under this condition, non-crosslinked components of the γ-secretase complex were reduced by >80% on immunoblotting. After centrifugation at 12,000 g , the supernatant was subjected to co-immunoprecipitation. RNA interference The following siRNA duplexes were purchased from Dharmacon (Lafayette, CO, USA): siGENOME SMART pool M-020514 for ILEI and D001210 for a non-targeting control. The M-020514 pool consisted of the four duplexes targeting the following sequences; F1: 5′-GAACAGCACAUAAAGAACA-3′; F2: 5′-GGAGAAGUAUUAGACACUA-3′; F3: 5′-GGAGCACAUCUAUUACUAA-3′; F4: 5′-GAACAAUAAGGAUACAAAC-3′. Cultured cells were transfected with individual or pooled siRNA duplexes using Lipofectamine RNAi MAX (Invitrogen). Secretase activity assays For a cell-free γ-secretase assay, cultured cells were homogenized in HEPES buffer (25 mM HEPES (pH 7.0), 150 mM NaCl, 5 mM MgCl 2 , 5 mM CaCl 2 , a protease inhibitor cocktail) and the postnuclear supernatants were centrifuged at 100,000 g for 1 h. The membrane pellets were lysed in 1% CHAPSO/HEPES buffer. Solubilized γ-secretase was recovered by centrifugation at 100,000 g for 30 min, and the concentrations of protein and CHAPSO were adjusted to 0.25 mg ml –1 and 0.25%, respectively. The resulting CHAPSO-solubilized γ-secretase was incubated with a recombinant APP-C99-Flag substrate for 6 h at 37 °C, and the Aβ40 and Aβ42 levels were measured by ELISA (WAKO Pure Chemical Industries, Osaka, Japan). For the NICD reporter assay, HEK293 cells in a 12-well plate were transiently transfected with NotchΔE (125 ng), HES-Y (125 ng) and 1.25 ng of the control Renilla luciferase reporter plasmid pRL-TK (Promega, Osaka, Japan). The cells were lysed 24 h after transfection, and firefly and Renilla luciferase activities were quantified using a dual luciferase reporter assay system (Promega) and a luminometer AB-2250 (Atto, Tokyo, Japan). β-Secretase activity of cell lysates was measured using a fluorometric reaction based on β-secretase cleavage of a synthetic substrate (R&D Systems). Organotypic brain culture Sagittal forebrain slices containing the hippocampus and cerebral cortex (400-μm thick) were prepared from 3-week-old female Wistar rats using a vibratome (Lancer Vibratome Series 1000, Vibratome, St Louis, MO, USA). The slices were cultured on semi-porous membrane inserts in six-well plates (0.4-μm pore diameter, Millipore) in a 37 °C, 5% CO 2 , 99% humidity incubator. The slices were maintained in standard medium consisting of DMEM Ham’s F12, 2% B27 neuronal supplement (Invitrogen) and antibiotic mixture (5 μg ml −1 penicillin, 5 μg ml −1 streptomycin and 10 μg ml −1 gentamycin). After 48 h, slices were treated with 10 ng ml −1 TGF-β1 (PeproTech, Rocky Hill, CT, USA) and rat ILEI-specific or non-targeting siRNA (Dharmacon) in Accell siRNA Delivery medium (Dharmacon) for another 48 h. Autopsy human brain tissues Frozen brain tissues from the frontal and temporal cortices of 15 patients with AD, 15 age-matched non-neurological disease control subjects and 10 non-AD neurological disease control subjects were obtained from the Brain Bank for Aging Research, Tokyo Metropolitan Institute of Gerontology (Tokyo, Japan). All the study subjects or their next of kin gave written informed consent for the brain donation, and the Shiga University of Medical Science Review Board approved the study protocol. All patients with AD fulfilled the National Institute of Neurological and Communicative Disorders and Stroke-Alzheimer’s Disease and Related Disorders Associations criteria for probable AD. Mice The Tg vector pMoPrP-ILEI was constructed by subcloning an Xho I– Xho I fragment of human ILEI cDNA into the Xho I site of the MoPrP vector that contains the mouse prion promoter to achieve neuron-specific expression [34] . Tg mice were generated by injection of linearized pMoPrP-ILEI DNA into fertilized C57BL/6 mouse oocytes using standard techniques. Tg founders were identified using PCR (see below). Five founders from each injection were backcrossed to C57BL/6 mice for one to two generations before protein and morphology analysis, and the two lines with the highest expression levels were retained for further experiments. The genotypes of Tg mice were determined by PCR using the following transgene-specific primer pair; mPrP-s 5′-CTGCTCCATTTTGCGTGACTC-3′ and hFAM3C-as 5′-CTTCCAGGCAGATTTTGGGTC-3′. APP-Tg (Tg2576) mice [33] were obtained from Taconic Farms (Hudson, NY, USA) and were bred by mating male mice with ILEI-Tg females. Female littermates were used in this study unless otherwise stated. All animal experiments were performed in accordance with national guidelines (Ministry of Education, Culture, Sports, Science, and Technology) and approved by the Shiga University of Medical Science Institutional Animal Care and Use Committees. Measurement of Aβ in mouse brains The right halves of mouse brains were homogenized using a motor-driven Teflon/glass homogenizer (ten strokes) in four volumes of Tris-buffered saline (20 mM Tris (pH 7.5), 150 mM NaCl, 0.5 mM EDTA) that contained a protease inhibitor cocktail. The homogenates were centrifuged at 100,000 g for 20 min on a TLA 100.4 rotor in a TLX ultracentrifuge (Beckman, Palo Alto, CA, USA). The supernatant was used as the soluble fraction. The pellet was lysed by brief sonication in an initial volume of 6 M guanidine hydrochloride in 50 mM Tris (pH 7.5), and then centrifuged at 100,000 g for 10 min. The supernatant was diluted at 1:12 and used as the insoluble fraction. The soluble and insoluble fractions were subjected to a DC protein assay (BioRad) and ELISA assays specific for mouse/rat Aβ40 and Aβ42 (IBL, Gunma, Japan) or for human Aβ40 and Aβ42 (WAKO Pure Chemical Industries). For quantification of Aβ plaque load on brain sections immunostained with anti-human Aβ (1:2,000, IBL), the number of and percentage area occupied by cortical and hippocampal plaques were measured on digital pictures with the ImageJ 1.46 program (National Institutes of Health, Bethesda, MD, USA). Immunohistochemistry The left halves of mouse brains were fixed in 4% paraformaldehyde in phosphate buffer. After blocking endogenous peroxidase activity, free-floating brain sections were incubated with appropriately diluted primary antibodies in PBS containing 2% BSA and 0.3% Triton-X100 at 4 °C overnight under horizontal agitation. Sections were then incubated with biotinylated secondary antibodies for 1 h. The immunoreactive products were visualized by incubating with 3,3′-diaminobenzidine containing nickel ammonium sulphate as an enhancing reagent. Stained sections were observed using a microscope (Olympus BX50, Tokyo, Japan). For double fluorescent immunostaining, sections were incubated with a mixture of rabbit polyclonal anti-ILEI antibody (1:4,000) and mouse monoclonal antibody against non-phosphorylated neurofilament (1:4,000, Covance), glial fibrillary acidic protein (1:4,000, Dako, Tokyo, Japan) or Iba1 (1:2,000, WAKO Pure Chemical Industries) overnight at 4 °C, then reacted with a mixture of secondary antibodies conjugated with Alexa488 (1:500, green) and Alexa594 (1:500, red) (Molecular Probes). The stained sections were analysed using a confocal laser-scanning microscope system (Digital Eclipse C1si-Ready, Nikon, Tokyo, Japan). Y-maze test The Y-maze apparatus consisted of three arms with grey walls (40 cm long, 10 cm wide, 10 cm high). The insides of the arms were identical, providing no intramaze cues. Each mouse was placed in the centre of the symmetrical Y-maze and was allowed to explore the maze freely for 8 min. The number and sequence of arms entered were recorded manually. The total number of arm entries was used to measure locomotor activity and motivation to explore the maze. The percentage of alternation, which was calculated by the proportion of alternations (an arm choice differing from the previous two choices) to the total number of alternation opportunities (total arm entries minus two), was used as a measure of spatial working memory. Experiments were done blind regarding the genotype of the mice. Statistical analysis Statistical evaluation was performed using two-tailed unpaired Student’s t -test unless otherwise stated. Data are presented as means±s.d. Statistical significance was defined at * P <0.05 or ** P <0.01. How to cite this article: Hasegawa, H. et al . The FAM3 superfamily member ILEI ameliorates Alzheimer’s disease-like pathology by destabilizing the penultimate amyloid-β precursor. Nat. Commun. 5:3917 doi: 10.1038/ncomms4917 (2014).